Lysine-specific demethylase 1 regulates differentiation onset and migration of trophoblast stem cells Propagation and differentiation of stem cell populations are tightly regulated to provide sufficient cell numbers for tissue formation while maintaining the stem cell pool. Embryonic parts of the mammalian placenta are generated from differentiating trophoblast stem cells (TSCs) invading the maternal decidua. Here we demonstrate that lysine-specific demethylase 1 (Lsd1) regulates differentiation onset of TSCs. Deletion of Lsd1 in mice results in the reduction of TSC number, diminished formation of trophectoderm tissues and early embryonic lethality. Lsd1 -deficient TSCs display features of differentiation initiation, including alterations of cell morphology, and increased migration and invasion. We show that increased TSC motility is mediated by the premature expression of the transcription factor Ovol2 that is directly repressed by Lsd1 in undifferentiated cells. In summary, our data demonstrate that the epigenetic modifier Lsd1 functions as a gatekeeper for the differentiation onset of TSCs, whereby differentiation-associated cell migration is controlled by the transcription factor Ovol2. During mammalian preimplantation development, the first two types of precursor cells to form are the inner cell mass (ICM) and the trophectoderm. The ICM further differentiates into primitive endoderm and the epiblast, the latter containing the progenitor cells that will form the embryo proper. Mural trophectoderm cells that are not in direct contact with the ICM differentiate early to form primary trophoblast giant cells mediating implantation of the blastocyst into the uterine wall shortly after embryonic day 3.5 (E3.5). Polar trophectoderm cells that directly overly the ICM give rise to trophoblast stem cells (TSCs) that are the cellular source for the embryonic part of the placenta. TSCs retain the capacity to self-renew and maintain an undifferentiated state that we refer to as stemness state. From E5.5, TSCs are found in extraembryonic ectoderm and until E9.5 in the chorionic ectoderm. Propagation of TSCs depends on Tgfβ and Fgf signals provided by the underlying epiblast, which are further enhanced by activities of feed-forward regulatory loops in the TSC compartment that also act on the epiblast [1] . Thus, trophoblast and epiblast propagation depend on reciprocal tissue crosstalk [2] . The extraembryonic ectoderm and at later stages the chorionic ectoderm provide TSCs that constitute the ectoplacental cone [3] , which will ultimately give rise to cells of the different placental lineages, syncytiotrophoblast, spongiotrophoblast and secondary trophoblast giant cells [2] , [3] . Multipotency and stemness of TSCs are characterized by the expression of a set of stem cell-associated transcription factors including caudal type homeobox2 (Cdx2) [4] and eomesodermin (Eomes) [5] , [6] . Loss-of-function studies have demonstrated crucial requirements of both factors for maintenance of TSCs in an undifferentiated state and downregulation of Cdx2 and Eomes denotes the loss of stem cell state [4] , [5] , [6] . Furthermore, TSC differentiation is accompanied by changes in cellular behaviour, such as increased cell size and acquisition of migration and invasion capacities required to form the embryonic–maternal interface of the placenta [7] . To date, little is known about cell autonomous mechanisms that repress premature TSC differentiation and differentiation-associated changes in cell behaviour. Recently, it became evident that chromatin-modifying enzymes function in tight cooperation with transcription factors to regulate stemness state and differentiation [8] . Epigenetic control mechanisms thus serve as an additional layer in the regulation of gene expression [9] , [10] , [11] , [12] . Acetylation, phosphorylation and methylation are reversible post-translational histone modifications. The methylation status of histone H3 at lysine 4 and 9 (H3K4 and H3K9, respectively) is linked to the expression level of the corresponding gene. While di- and trimethylated H3K4 (H3K4me3/2) are so-called ‘active chromatin marks’ associated with active transcription, di- and trimethylated H3K9 (H3K9me3/2) are denoted transcriptionally ‘repressive marks’ [9] . We and others have shown that lysine-specific demethylase 1 (Lsd1; also known as Kdm1a, Aof2) selectively removes mono- and dimethyl groups from H3K4 or H3K9, thereby causing either repression or activation of gene transcription [13] , [14] , [15] , [16] , [17] , [18] , [19] . Several studies have reported that Lsd1 -deficient mouse embryos die prior to gastrulation at E7.5 (refs 19 , 20 , 21 , 22 ) proposing predominant functions in pluripotent cells of the epiblast. Analysis of Lsd1 -deficient mouse embryonic stem cells in culture suggested a progressive loss of DNA methylation [19] , altered expression of genes crucial for ES cell differentiation [21] or a bias towards extraembryonic lineage differentiation [20] . Furthermore, Adamo et al. [23] reported that LSD1 regulates the balance between self-renewal and differentiation of human ESCs (hESCs). In contrast, analyses of Lsd1 functions in other stem cell compartments of the early embryo, including functional studies in TSCs, have remained elusive. Here we analyse Lsd1 -deficient pregastrulation-stage mouse embryos and observe previously unrecognized defects in the trophectoderm lineage. The trophectoderm-specific deletion of Lsd1 leads to a significant reduction in the extraembryonic ectoderm, indicating an intrinsic requirements of Lsd1 function for trophectoderm development. We define the transcription factor ovol-like 2 ( Ovol2 ) as a directly repressed Lsd1 target gene, thereby inhibiting premature cell migration and invasion. In conclusion, our data reveal that the epigenetic modifier Lsd1 acts as a crucial coordinator of trophoblast development by inhibiting premature differentiation onset accompanied with increased cell migration. Differential requirements of Lsd1 Several studies have reported functions of Lsd1 in ESCs and in the early epiblast [19] , [20] , [21] , [22] , [23] , [24] . Whether or not absence of Lsd1 in the epiblast indeed accounts for the early embryonic lethality of Lsd1 -deficient embryos preceding E7.5 has not been conclusively addressed. To specifically dissect Lsd1 functions in the different cell lineages of the pregastrula stage mouse embryo, we engineered a novel conditional Lsd1 allele by flanking exon 1 with loxP sites. In agreement with earlier reports [19] , [20] , [21] , [22] , ubiquitous deletion of the conditional Lsd1 allele ( Lsd1 −/− ) leads to early embryonic lethality, and only resorbed embryos are detected by E7.5 ( Fig. 1a ). To evaluate tissue-restricted functions, we deleted Lsd1 by crossing the conditional Lsd1 allele to the well-described transgenic Sox2.Cre deleter strain [25] , which robustly mediates Cre recombination specifically in the early post-implantation epiblast ( Lsd1 Sox2-Cre ) but not in the extraembryonic lineages. Immunofluorescence staining confirms epiblast-specific deletion of Lsd1 while expression is maintained in other tissues, namely the visceral endoderm and the extraembryonic ectoderm ( Fig. 1b ). Unexpectedly, epiblast-specific deletion of Lsd1 delays the early lethal phenotype of ubiquitous Lsd1 −/− embryos ( Fig. 1a ), and Lsd1 Sox2-Cre embryos appear grossly normal at E7.5. Further development of Lsd1 Sox2-Cre embryos is arrested shortly after gastrulation onset and they do not undergo embryonic turning at E8.5. Besides the developmental block at later stages, our results demonstrate a remarkably normal development of Lsd1 Sox2-Cre embryos until midgastrulation, suggesting additional functions of Lsd1 within the extraembryonic lineages. Consequently, we specifically deleted Lsd1 in TSCs of the extraembryonic ectoderm using an Eomes Cre deleter strain ( Lsd1 Eomes-Cre ) [26] , where Cre is active in TSCs from early post-implantation stages onwards ( Fig. 1b ). Mutant embryos develop beyond gastrulation ( Fig. 1a,b ) but show severe morphological abnormalities at E7.5 ( Fig. 1a ) with development arrest before E8.5. 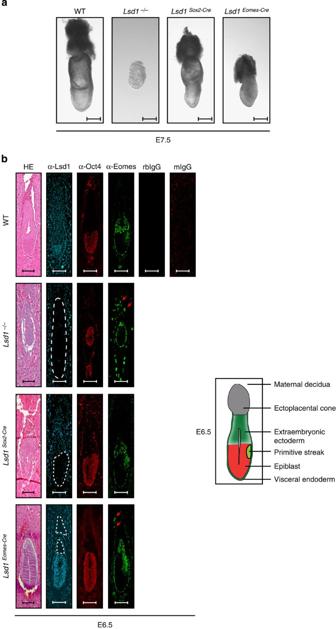Figure 1:Lsd1−/−embryos and trophoblast-specific deletion of Lsd1 exhibit pronounced trophectoderm defects. (a) Representative morphology of whole-mount wild-type (WT), constitutively deleted (Lsd1−/−), epiblast-specific (Lsd1Sox2-Cre) and trophoblast-specificLsd1-deficient (Lsd1Eomes-Cre) embryos at E7.5. (b) Comparison of histological sections of WT,Lsd1−/−,Lsd1Sox2-CreandLsd1Eomes-CreE6.5 embryos by HE staining, immunofluorescence with indicated antibodies and the corresponding IgG controls. Dashed lines circle theLsd1-deficient parts of the embryos. Arrows indicate ectopic, Eomes-positive cells outside of the region of the extraembryonic ectoderm. The cartoon is depicting the different cell lineages of the E6.5 embryo. Scale bars represent 200 μm (a) and 100 μm (b). Figure 1: Lsd1 −/− embryos and trophoblast-specific deletion of Lsd1 exhibit pronounced trophectoderm defects. ( a ) Representative morphology of whole-mount wild-type (WT), constitutively deleted ( Lsd1 −/− ), epiblast-specific ( Lsd1 Sox2-Cre ) and trophoblast-specific Lsd1 -deficient ( Lsd1 Eomes-Cre ) embryos at E7.5. ( b ) Comparison of histological sections of WT, Lsd1 −/− , Lsd1 Sox2-Cre and Lsd1 Eomes-Cre E6.5 embryos by HE staining, immunofluorescence with indicated antibodies and the corresponding IgG controls. Dashed lines circle the Lsd1 -deficient parts of the embryos. Arrows indicate ectopic, Eomes-positive cells outside of the region of the extraembryonic ectoderm. The cartoon is depicting the different cell lineages of the E6.5 embryo. Scale bars represent 200 μm ( a ) and 100 μm ( b ). Full size image Thus, in comparison to constitutive Lsd1 -deficient embryos, specific deletion in either the epiblast or the trophectoderm leads to less pronounced phenotypes demonstrating requirements of Lsd1 in both compartments for normal embryonic development. Deletion of Lsd1 impairs trophectoderm development To further delineate functions of Lsd1 in the different tissues of the early embryo, we performed histological analysis of wild-type, Lsd1 −/− , Lsd1 Sox2-Cre and Lsd1 Eomes-Cre embryos at E6.5 ( Fig. 1b for schematic of the different embryonic cell types). Consistent with previous reports [19] , [20] , [21] , [22] , we find that Lsd1 −/− embryos are significantly reduced in size but possess cells of the three early embryonic lineages, namely epiblast, extraembryonic ectoderm and primitive endoderm/visceral endoderm as shown by haematoxylin and eosin (HE) staining ( Fig. 1b ). Accordingly, immunofluorescence analysis shows similar expression of the pluripotency-associated marker Oct4 (also known as Pou5f1) [27] in the epiblast of wild-type and Lsd1 −/− embryos ( Fig. 1b ; Supplementary Fig. 1a ). To reveal the presence of trophectoderm and visceral endoderm, we used antibody staining for Eomes, which is a marker for TSCs and embryonic visceral endoderm cells [28] . Expression of Oct4 and Eomes indicates the presence of all three lineages in Lsd1 −/− embryos; however, in comparison to wild-type embryos we observed a striking reduction of Eomes- and Cdx2-positive TSCs in the extraembryonic ectoderm ( Fig. 1b ; Supplementary Fig. 1a,b ). To analyse whether the reduced number of Eomes-expressing TSCs is a secondary effect due to the loss of Lsd1 in the epiblast, or whether this resembles an autonomous effect of Lsd1 depletion in the trophectoderm, we analysed Lsd1 Sox2-Cre and Lsd1 Eomes-Cre embryos. While deletion of Lsd1 from the epiblast ( Lsd1 Sox2-Cre ) does not compromise the trophectoderm compartment, deletion of Lsd1 in the trophectoderm ( Lsd1 Eomes-Cre ) leads to a markedly reduced size of the extraembryonic ectoderm, similar to the constitutive Lsd1 −/− mutant embryos ( Fig. 1b ). Interestingly, we consistently observed ectopic, Eomes-expressing cells that were detached from the extraembryonic ectoderm and showed enlarged cell size in Lsd1 −/− embryos. These types of cells could also be found in Lsd1 Eomes-Cre trophectoderm-specific mutants, albeit at reduced frequency, whereas similar observations were not made in wild-type or Lsd1 Sox2-Cre embryos ( Fig. 1b ). Lsd1 regulates differentiation of TSCs TSCs can be efficiently differentiated into derivatives of the trophectoderm, namely syncytiotrophoblast, spongiotrophoblast and trophoblast giant cells in culture [2] . To test for the differentiation potential of Lsd1 −/− TSCs, we used a cell culture system as the corresponding in vitro correlate [29] . TSCs were isolated from E3.5 blastocysts harbouring either a transgenic doxycyclin (Dox)-inducible RNA interference construct ( Lsd1 iKD ) or the tamoxifen (Tx)-inducible CreER T2 -recombinase combined with the Lsd1 conditional alleles to inducibly delete Lsd1 ( Lsd1 iKO ). Drug administration leads to the loss of Lsd1 protein by day 8 in iKO and day 4 in iKD cells as shown using western blot analyses ( Fig. 2a ). Of note, all experiments were performed with several independent iKD and iKO TSCs excluding that clonal variations account for observed phenotypes. For simplicity, only data from iKO cells are shown in following analyses, if not otherwise indicated. We first treated Lsd1 iKO cells for 8 days with Tx prior to induction of differentiation by the removal of FGF4 and mouse embryonic fibroblast (MEF)-conditioned medium. As expected, differentiation leads to rapid downregulation of TSC stemness marker genes such as Cdx2 and Eomes in both Lsd1 −/− and wild-type control cells ( Fig. 2b ). Concomitantly, marker genes for differentiating trophectoderm become upregulated from day 2 of differentiation ( Fig. 2b ). Interestingly, the differentiation behaviour of wild-type and Lsd1 −/− cells exhibits striking differences. While Lsd1 −/− cells show a significant increase in expression of the syncytiotrophoblast marker Gcm1 , spongiotrophoblast markers Mash2 and Tpbpa are significantly reduced compared with the wild type ( Fig. 2b ). Similarly, the trophoblast giant cell markers Pl1 , Pl2 (also known as Prl3d1 and Prl3b1 , respectively) and Plf (also known as Prl2c2 ) are drastically reduced or absent in Lsd1 −/− cells while they become abundantly expressed in differentiating Lsd1 -proficient TSCs ( Fig. 2b ; Supplementary Fig. 2a,b ). Of note, Tx treatment does not alter the differentiation behaviour of wild-type TSCs ( Supplementary Fig. 2c ). We therefore conclude that the loss of Lsd1 impairs differentiation towards spongiotrophoblast and secondary giant cells in favour of syncytiotrophoblast. 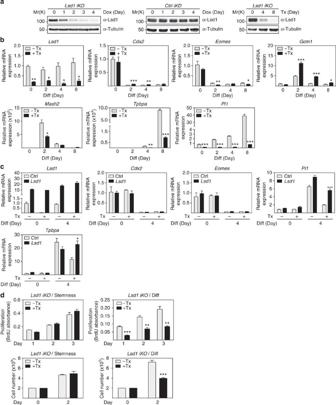Figure 2: Lsd1 regulates differentiation of TSCs. (a) Efficiency ofLsd1knockdown (Lsd1 iKD) and Cre-mediated genetic deletion (Lsd1 iKO) in TSCs is analysed using western blot. Cells were treated with Dox or Tx for the indicated duration. Specificity ofLsd1knockdown is verified using TSCs expressing short hairpin RNA directed against LacZ (Ctrl iKD). Tubulin is used as a loading control. (b) qRT–PCR analyses of mRNA expression levels ofLsd1and indicated lineage markers during differentiation inLsd1 iKOTSCs in the absence or presence of Tx. (c) The expression levels of indicated genes iniKOTSCs transfected with anLsd1-expression vector (Lsd1), or an empty vector (Ctrl) is monitored during differentiation by qRT–PCR in the absence or presence of Tx. (d) Proliferation assays ofLsd1 iKOTSCs in stemness and differentiation (Diff) conditions in the absence or presence of Tx determined by BrdU incorporation (upper panel) or by cell number using FACS (lower panel). qRT–PCR data are normalized toGapdhand represented as mean+s.e.m. Experiments (b–d) were independently repeated at least three times in triplicate. Statistical analysis was performed using two-tailed Student’st-test. *P<0.05; **P<0.01; ***P<0.001. Figure 2: Lsd1 regulates differentiation of TSCs. ( a ) Efficiency of Lsd1 knockdown ( Lsd1 iKD ) and Cre-mediated genetic deletion ( Lsd1 iKO ) in TSCs is analysed using western blot. Cells were treated with Dox or Tx for the indicated duration. Specificity of Lsd1 knockdown is verified using TSCs expressing short hairpin RNA directed against LacZ ( Ctrl iKD ). Tubulin is used as a loading control. ( b ) qRT–PCR analyses of mRNA expression levels of Lsd1 and indicated lineage markers during differentiation in Lsd1 iKO TSCs in the absence or presence of Tx. ( c ) The expression levels of indicated genes in iKO TSCs transfected with an Lsd1 -expression vector ( Lsd1 ), or an empty vector (Ctrl) is monitored during differentiation by qRT–PCR in the absence or presence of Tx. ( d ) Proliferation assays of Lsd1 iKO TSCs in stemness and differentiation (Diff) conditions in the absence or presence of Tx determined by BrdU incorporation (upper panel) or by cell number using FACS (lower panel). qRT–PCR data are normalized to Gapdh and represented as mean+s.e.m. Experiments ( b – d ) were independently repeated at least three times in triplicate. Statistical analysis was performed using two-tailed Student’s t -test. * P <0.05; ** P <0.01; *** P <0.001. Full size image To further confirm requirements of Lsd1 for TSC differentiation, we reintroduced Lsd1 into Lsd1 iKO TSCs and examined the expression of stem cell and differentiation markers in the absence or presence of Tx. As expected, expression levels of the stem cell markers Cdx2 and Eomes are not significantly affected, while transcription of the syncytiotrophoblast, spongiotrophoblast and giant cell marker genes Pl1 , Tpbpa , Plf and Gcm1 , respectively, are restored to wild-type levels, demonstrating that the phenotype of Lsd1 −/− cells can be rescued by ectopic expression of Lsd1 ( Fig. 2c ; Supplementary Fig. 2d,e ). Next, we addressed whether the demethylase activity of Lsd1 is required for directing TSC fate by ectopic expression of a catalytic inactive mutant of Lsd1 (Lsd1 Mut ) [30] . Ectopic expression of the Lsd1 mutant protein in Lsd1 −/− TSCs does not alter the transcription of stem cell-associated genes such as Eomes ( Supplementary Fig. 2d ). Unlike wild-type Lsd1, the enzymatic inactive protein fails to restore the transcription of trophoblast differentiation markers such as Plf to wild-type levels ( Supplementary Fig. 2d ). We therefore conclude that the enzymatic activity of Lsd1 plays a decisive role in controlling the lineage decisions of differentiating TSCs. To quantitatively assess whether there are differences in the proliferation of wild-type and Lsd1 −/− TSCs, we performed BrdU incorporation assays. Under stemness-maintaining conditions, Lsd1 -proficient and Lsd1 -deficient cells do not show significant differences in proliferation ( Fig. 2d ). However, when TSCs are induced to differentiate, we observe significantly reduced proliferation rates of Lsd1 −/− cells ( Fig. 2d ). To distinguish between endoreduplication of trophoblast giant cells and cell proliferation, we performed a second DNA content-independent assay. Determination of the cell number by FACS before and during differentiation corroborated the decrease in proliferation specifically in differentiating Lsd1 -deficient TSCs ( Fig. 2d ). The reduced proliferation of differentiated Lsd1 −/− TSCs may account, at least in part, for the overall decrease in trophectoderm tissue in Lsd1 −/− embryos. Lsd1 restrains migration and invasion of TSCs The analysis of cell morphology and cellular behaviour revealed striking changes in both iKO and iKD Lsd1 -depleted TSCs in comparison to control cultures ( Fig. 3 ). Typically, wild-type undifferentiated TSCs are characterized by the formation of dense epithelial colonies with hardly visible cell borders and relatively small cell size. In contrast, upon depletion of Lsd1 , the cell size of TSCs is markedly increased, and the morphology of the colonies is less compact with clearly discernable cell borders ( Fig. 3a ). These features are usually associated with the early onset of TSC differentiation (Day 2; Fig. 3a ). FACS-assisted cell size analyses revealed enlargement of Lsd1 −/− TSCs similar to the size increase of wild-type TSCs on day 2 of differentiation ( Fig. 3b ). Additionally, phalloidin staining of the cytoskeleton reveals increased spreading of Lsd1 −/− -TSCs ( Supplementary Fig. 3a ). However, despite the fact that Lsd1 −/− TSCs lose their characteristic morphology, they maintain expression of stemness-associated markers Cdx2 and Eomes ( Fig. 2b ). 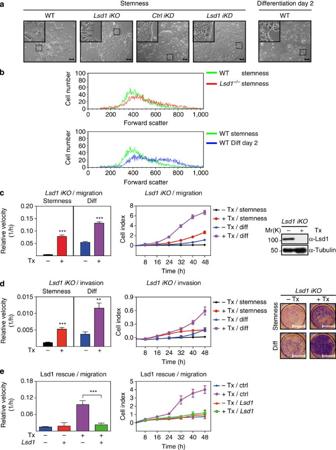Figure 3: Lsd1 restrains migration and invasion of TSCs. (a) Representative images of TSC colonies showing the morphology of WT,Lsd1 iKO,Ctrl iKDandLsd1 iKDTSCs after administration of Tx or Dox for 8 days in stemness conditions in comparison to WT TSCs after 2 days of differentiation. Scale bars represent 100 μm. (b) FACS analyses of cell size of wild-type TSCs on day 0 (green), day 2 (blue) andLsd1−/−TSCs (red). (c) Migration assays ofLsd1 iKOTSCs in the absence or presence of Tx under stemness or differentiation (Diff) conditions recorded in real time. Depletion of Lsd1 iniKOcells is controlled using western blot. Tubulin is used as a loading control. (d) 3D-matrix invasion assays ofLsd1 iKOTSCs in the absence or presence of Tx under stemness or differentiation (Diff) conditions recorded in real time. Cells that invaded the matrix and reached the lower surface of the transwell filter are stained by crystal violet. Scale bars represent 3 mm. (e) Migration assays of undifferentiatedLsd1 iKOTSCs transfected with an Lsd1-expression plasmid (Lsd1) or an empty vector (Ctrl) in the absence or presence of Tx demonstrate that Lsd1 expression rescues increased migration of Lsd1 iKO cells. Bars represent mean±s.e.m. or +s.e.m. Experiments (c–e) were independently repeated at least three times in triplicate. Statistical analysis was performed using two-tailed Student’st-test. **P<0.01; ***P<0.001. Figure 3: Lsd1 restrains migration and invasion of TSCs. ( a ) Representative images of TSC colonies showing the morphology of WT, Lsd1 iKO , Ctrl iKD and Lsd1 iKD TSCs after administration of Tx or Dox for 8 days in stemness conditions in comparison to WT TSCs after 2 days of differentiation. Scale bars represent 100 μm. ( b ) FACS analyses of cell size of wild-type TSCs on day 0 (green), day 2 (blue) and Lsd1 −/− TSCs (red). ( c ) Migration assays of Lsd1 iKO TSCs in the absence or presence of Tx under stemness or differentiation (Diff) conditions recorded in real time. Depletion of Lsd1 in iKO cells is controlled using western blot. Tubulin is used as a loading control. ( d ) 3D-matrix invasion assays of Lsd1 iKO TSCs in the absence or presence of Tx under stemness or differentiation (Diff) conditions recorded in real time. Cells that invaded the matrix and reached the lower surface of the transwell filter are stained by crystal violet. Scale bars represent 3 mm. ( e ) Migration assays of undifferentiated Lsd1 iKO TSCs transfected with an Lsd1-expression plasmid ( Lsd1 ) or an empty vector (Ctrl) in the absence or presence of Tx demonstrate that Lsd1 expression rescues increased migration of Lsd1 iKO cells. Bars represent mean±s.e.m. or +s.e.m. Experiments ( c – e ) were independently repeated at least three times in triplicate. Statistical analysis was performed using two-tailed Student’s t -test. ** P <0.01; *** P <0.001. Full size image To explore whether the change in cell morphology of Lsd1 -deficient TSCs is reflected by functional differences in cell behaviour, we performed migration and invasion assays using a transwell system in real time. TSCs were either kept under stemness conditions or induced to differentiate during the course of the experiment. Interestingly, Lsd1 −/− TSCs maintained under stemness conditions already show a significant increase in cell migration ( Fig. 3c ) and invasion ( Fig. 3d ), which is further enhanced under differentiation conditions ( Fig. 3c,d ). To control for specificity, we treated Lsd1-proficient wild-type TSCs with Tx, which does not alter migration ( Supplementary Fig. 3b ). Importantly, reintroducing Lsd1 rescues the elevated migration of Lsd1 −/− TSCs ( Fig. 3e ). To determine whether the demethylase activity of Lsd1 accounts for the observed migration phenotype, we additionally performed migration analysis of wild-type TSC in the presence of specific Lsd1 inhibitors [31] , [32] . Similar to the deletion of Lsd1 , inhibitor treatment causes a significant increase in TSC migration indicating that the enzymatic activity of Lsd1 is essential ( Supplementary Fig. 3c ). In agreement, the introduction of an enzymatic inactive Lsd1 mutant does not rescue the migration phenotype of Lsd1 −/− TSCs ( Supplementary Fig. 3d ). Thus, the epigenetic regulator Lsd1 represses the migration of TSCs in culture, potentially also explaining the appearance of Eomes-expressing trophoblast cells outside the extraembryonic ectoderm in Lsd1 -deficient embryos. Deletion of Lsd1 lowers the threshold for differentiation onset To identify potential Lsd1 target genes that have an impact on the behavioural changes of Lsd1-depleted TSCs, we performed transcriptional profiling by microarrays in the presence or absence of Lsd1. RNA was collected on day 0 (TSCs under stemness conditions), day 2 and day 4 after induction of differentiation. We first analysed Lsd1-dependent gene expression by comparison of transcription in Lsd1 -proficient and Lsd1 −/− TSCs at all three time points. In total, the expression of ∼ 1,000 genes is altered (analysis of variance test, P -value <10 −5 and more than twofold expression change) ( Fig. 4a ). In the absence of Lsd1, roughly 700 genes show increased expression while the transcription of 300 genes is decreased, demonstrating that the majority of target genes is repressed by Lsd1. Analyses of gene ontology and signalling pathways did not reveal any significant signature ( Supplementary Tables 1,2 ). Based on our previous results, we hypothesized that Lsd1 depletion under stemness conditions alters the characteristics of TSCs towards an early-onset-differentiated phenotype. Therefore, we compared the gene expression profiles during differentiation (wild-type TSCs day 0 versus day 2 of differentiation) with the differentially expressed genes after Lsd1 deletion ( Lsd1 −/− TSCs versus wild-type TSCs under stemness conditions; Supplementary Table 3 ). Importantly, 52 genes associated with the differentiation of wild-type TSCs between day 0 and day 2 are already prematurely differentially expressed in Lsd1 −/− cells under stemness-maintaining conditions (day 0; Fig. 4b ). This group comprises 26% (52 of 198) of all genes regulated by Lsd1 under stemness conditions. This proportion increases to 39% (78 of 198) when those genes are compared that are differentially regulated during TSC differentiation between day 0 and day 4 ( Fig. 4b ). 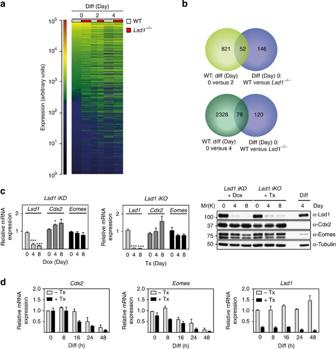Figure 4: Premature differential expression of differentiation-associated genes inLsd1-deficient TSCs. (a) Comparative expression heat map of WT andLsd1 iKOTSCs under stemness and differentiation conditions shows all significantly Lsd1-regulated genes. (b) Venn diagrams showing the overlap of differentially expressed genes in WT andLsd1 iKOTSCs under stemness conditions (purple) and genes that are differentially expressed in WT TSCs after 2 (bright green) and 4 (dark green) days of differentiation. (c) Comparison of mRNA and protein expression levels of Lsd1 and the stemness markersCdx2andEomesby qRT–PCR and western blot inLsd1 iKDandLsd1 iKOTSCs treated with Dox or Tx for the indicated time points. Wild-type TSCs induced to differentiate for 4 days are used as differentiation (Diff) control and tubulin as loading control. (d) qRT–PCR analyses of mRNA expression levels ofLsd1and indicated lineage markers during early time points of differentiation inLsd1 iKOTSCs in the absence or presence of Tx. qRT–PCR data are normalized toGapdhand represented as mean+s.e.m. Experiments (c,d) were independently repeated at least three times in triplicate. Statistical analysis was performed using analysis of variance (a) and two-tailed Student’st-test (b–d). ***P<0.001. Figure 4: Premature differential expression of differentiation-associated genes in Lsd1 -deficient TSCs. ( a ) Comparative expression heat map of WT and Lsd1 iKO TSCs under stemness and differentiation conditions shows all significantly Lsd1-regulated genes. ( b ) Venn diagrams showing the overlap of differentially expressed genes in WT and Lsd1 iKO TSCs under stemness conditions (purple) and genes that are differentially expressed in WT TSCs after 2 (bright green) and 4 (dark green) days of differentiation. ( c ) Comparison of mRNA and protein expression levels of Lsd1 and the stemness markers Cdx2 and Eomes by qRT–PCR and western blot in Lsd1 iKD and Lsd1 iKO TSCs treated with Dox or Tx for the indicated time points. Wild-type TSCs induced to differentiate for 4 days are used as differentiation (Diff) control and tubulin as loading control. ( d ) qRT–PCR analyses of mRNA expression levels of Lsd1 and indicated lineage markers during early time points of differentiation in Lsd1 iKO TSCs in the absence or presence of Tx. qRT–PCR data are normalized to Gapdh and represented as mean+s.e.m. Experiments ( c , d ) were independently repeated at least three times in triplicate. Statistical analysis was performed using analysis of variance ( a ) and two-tailed Student’s t -test ( b – d ). *** P <0.001. Full size image The altered expression of genes associated with early differentiation confirmed our hypothesis that Lsd1 −/− TSCs lose stem cell characteristics. However, under stemness-maintaining conditions, Cdx2 and Eomes expression is similar in Lsd1 -depleted and Lsd1 -proficient TSCs ( Fig. 4c ). This raises the question whether Lsd1 −/− TSCs might initiate the differentiation onset faster than wild-type cells upon removal of stem cell-maintaining conditions. To validate this hypothesis, we quantified the transcription of TSC marker genes during the first hours of differentiation. Upon induction of differentiation, the transcription of both stem cell marker genes is reduced considerably faster in Lsd1 -deficient TSCs implying that the deletion of Lsd1 lowers the threshold for differentiation onset ( Fig. 4d ). The fact that Lsd1 -depleted TSCs show characteristics of early differentiation ( Figs 3 and 4d ) suggests that the group of prematurely differentially expressed genes in Lsd1 −/− cells contains Lsd1 targets that have an impact on cellular morphology and behaviour such as migration. Lsd1 controls expression of Ovol2 in TSCs and trophectoderm Next, we aimed to identify Lsd1-regulated genes that mediate the effect of Lsd1 depletion on increased TSC migration. First, we validated our microarray analysis via quantitative reverse transcription–PCR (qRT–PCR) by choosing Lsd1 and known markers of trophoblast stemness and differentiation such as Cdx2 and Pl1 and Pl2 , in addition to selected differentially expressed genes ( Fig. 2b ; Supplementary Fig. 2a ). From our list of confirmed differentially expressed genes ( Supplementary Fig. 4 ), we consequently focused on genes with potential functions in cell migration. Combining data of our expression profiles with published expression patterns and reports on gene-function, we identified the zinc-finger transcription factor Ovol2 as a promising candidate. Ovol2 expression is first found in cells of the chorionic plate and later within the labyrinthine layer of the developing placenta [33] . Targeted deletion of Ovol2 leads to embryonic death from E9.5 with a pronounced phenotype of the placenta, characterized by a lack of an elaborated labyrinthine layer [33] . Furthermore, it was suggested that Ovol2 is involved in the migration of neural crest derivatives [34] . Using qRT–PCR, western blot analyses and a polymerase II chromatin immunoprecipitation (ChIP) we confirmed the dynamic expression of Ovol2 during TSC differentiation ( Fig. 5a,b ; Supplementary Fig. 5a ). While Ovol2 expression is low in Lsd1 -proficient TSCs under stemness conditions, there is a continuous and robust increase in expression during TSC differentiation. In Lsd1 −/− TSCs, the expression of Ovol2 is prematurely increased under stemness conditions and during early stages of differentiation, while the differences in RNA and protein levels between control and Lsd1 -deficient TSCs equal during late differentiation ( Fig. 5a,b ). Re-introduction of Lsd1 in Lsd1 −/− TSCs restored Ovol2 transcription and protein levels ( Supplementary Fig. 5b ). 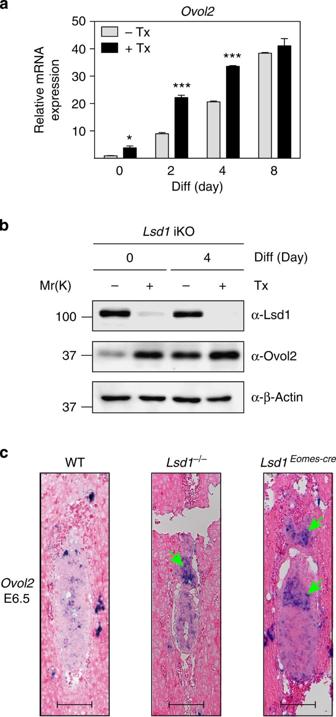Figure 5: Lsd1 represses expression of Ovol2 in TSCs and in the trophectoderm. (a) qRT–PCR analyses of mRNA expression levels ofOvol2during differentiation ofLsd1 iKOTSCs in the absence or presence of Tx. (b) Western blot analyses of Lsd1 and Ovol2 protein levels inLsd1 iKOTSCs on days 0 and 4 of differentiation in the presence or absence of Tx. Beta actin is used as loading control. (c)In situhybridization using anOvol2probe at E6.5 in WT,Lsd1−/−andLsd1Eomes-Creembryos. Arrows indicate ectopicOvol2expression. Scale bars represent 100 μm. qRT–PCR data are normalized toGapdhand are represented as mean+s.e.m. Experiment (a) was independently repeated at least three times in triplicate. Statistical analysis was performed using two-tailed Student’st-test. *P<0.05; ***P<0.001. Figure 5: Lsd1 represses expression of Ovol2 in TSCs and in the trophectoderm. ( a ) qRT–PCR analyses of mRNA expression levels of Ovol2 during differentiation of Lsd1 iKO TSCs in the absence or presence of Tx. ( b ) Western blot analyses of Lsd1 and Ovol2 protein levels in Lsd1 iKO TSCs on days 0 and 4 of differentiation in the presence or absence of Tx. Beta actin is used as loading control. ( c ) In situ hybridization using an Ovol2 probe at E6.5 in WT, Lsd1 −/− and Lsd1 Eomes-Cre embryos. Arrows indicate ectopic Ovol2 expression. Scale bars represent 100 μm. qRT–PCR data are normalized to Gapdh and are represented as mean+s.e.m. Experiment ( a ) was independently repeated at least three times in triplicate. Statistical analysis was performed using two-tailed Student’s t -test. * P <0.05; *** P <0.001. Full size image To assess whether Ovol2 expression is similarly changed in vivo in Lsd1 -deficient trophectoderm, we performed in situ hybridization analysis of histological sections from wild-type, Lsd1 −/− and Lsd1 Eomes-Cre embryos at E6.5. In wild-type embryos, Ovol2 is expressed in syncytiotrophoblast cell from E8 ( Supplementary Fig. 5c ) with no Ovol2 expression in embryonic or extraembryonic regions of the wild-type conceptus at E6.5 ( Fig. 5c ). In striking contrast, we find abundant expression of Ovol2 within the extraembryonic compartments of Lsd1 −/− and of Lsd1 Eomes-Cre embryos prematurely at E6.5 ( Fig. 5c ). Thus, deletion of Lsd1 leads to premature expression of Ovol2 in cultured TSCs and in embryos. Lsd1 directly suppresses Ovol2 expression in TSCs To investigate whether Lsd1 directly regulates and occupies the Ovol2 promoter, we performed ChIP using an Lsd1-specific antibody followed by qPCR for genomic regions of the Ovol2 gene locus. Lsd1 specifically binds to a distal promoter region 1.3 kb upstream to the transcription start site (TSS) and around the TSS of the Ovol2 gene ( Fig. 6a ; Supplementary Fig. 6a ). Binding of Lsd1 is specific since using an IgG control or performing ChIP in Lsd1 −/− cells fails to enrich chromatin ( Fig. 6 ; Supplementary Fig. 6a ). To further control for specificity we analysed an unrelated region 4.6 kb upstream of the TSS that is not occupied by Lsd1 ( Fig. 6a ; Supplementary Fig. 6a,c ). To analyse whether Lsd1 represses Ovol2 transcription by the removal of mono- and dimethyl H3K4 marks at the Ovol2 promoter, we performed ChIP with methyl-specific antibodies and compared the methylation levels of wild-type and Lsd1 −/− TSCs. Consistent with increased Ovol2 expression in Lsd1 −/− TSCs ( Fig. 5a,b ; Supplementary Fig. 5a ), levels of H3K4 methyl marks are increased in Lsd1 −/− TSCs ( Fig. 6b ; Supplementary Fig. 6b,d ) suggesting that Lsd1 demethylates H3K4me2/1. Interestingly, H3K9 methylation levels are generally low at the Ovol2 promoter and during TSC differentiation the overall amount of H3K4me3 does not increase ( Fig. 6b ; Supplementary Fig. 6b,d ), indicating that additional chromatin modifiers might contribute to the transcriptional regulation of Ovol2 . Consistent with this hypothesis we observe a decrease in the repressive H3K27me3 mark at the Ovol2 promoter during differentiation ( Fig. 6b ; Supplementary Fig. 6b ). Importantly, on day 4 of TSC differentiation, Lsd1 does no longer bind to the Ovol2 promoter ( Fig. 6b ), despite abundant expression of Lsd1 throughout differentiation ( Fig. 2b ; Supplementary Fig. 2b,c ). Consequently, no significant differences in the levels of methylated H3K4 and H3K9 between Lsd1 -proficient and Lsd1 −/− TSCs are detected during differentiation ( Fig. 6b ; Supplementary Fig. 6b ). In summary, our data suggest that Lsd1 represses Ovol2 expression in undifferentiated TSCs by binding to its promoter. In contrast, in differentiating TSCs Lsd1 is not associated with the promoter and consequently does no longer prevent Ovol2 expression, despite persistent Lsd1 protein levels. 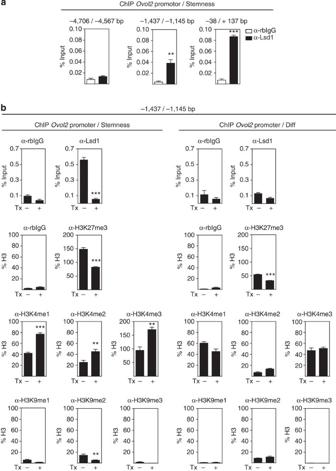Figure 6: Lsd1 directly regulatesOvol2transcription in undifferentiated TSCs. (a) ChIP experiments are performed with Lsd1 antibodies and IgG to detect Lsd1-specific binding at the distal promoter region (−1,437 bp/−1,145 bp) and the transcription start site (−38 bp/+137 bp) ofOvol2compared with a control region (−4,706 bp/−4,567 bp). (b) ChIP experiments are performed with the indicated antibodies to detect associated changes of chromatin marks at theOvol2promoter (−1,437 bp/−1,146 bp). ChIP is performed usingLsd1 iKOTSCs in the presence or absence of Tx under stemness conditions and after 4 days of differentiation. Bars are represented as mean+s.e.m. Experiments were independently repeated at least three times in triplicate. Statistical analysis was performed using two-tailed Student’st-test. **P<0.01; ***P<0.001. Figure 6: Lsd1 directly regulates Ovol2 transcription in undifferentiated TSCs. ( a ) ChIP experiments are performed with Lsd1 antibodies and IgG to detect Lsd1-specific binding at the distal promoter region (−1,437 bp/−1,145 bp) and the transcription start site (−38 bp/+137 bp) of Ovol2 compared with a control region (−4,706 bp/−4,567 bp). ( b ) ChIP experiments are performed with the indicated antibodies to detect associated changes of chromatin marks at the Ovol2 promoter (−1,437 bp/−1,146 bp). ChIP is performed using Lsd1 iKO TSCs in the presence or absence of Tx under stemness conditions and after 4 days of differentiation. Bars are represented as mean+s.e.m. Experiments were independently repeated at least three times in triplicate. Statistical analysis was performed using two-tailed Student’s t -test. ** P <0.01; *** P <0.001. Full size image Ovol2 induces migration and invasion of Lsd1 −/− TSCs Since we observe increased and aberrant migration and invasion of Lsd1 -deficient TSCs, we asked whether prematurely expressed Ovol2 accounts for the pro-migratory phenotype. We ectopically expressed Ovol2 in wild-type TSCs and measured migration and invasion in real time. Intriguingly, Ovol2 overexpression induces increased TSC migration ( Fig. 7a ) and invasion ( Fig. 7b ) and thus strikingly phenocopies the behaviour of Lsd1 −/− TSCs. To address whether Ovol2 is the predominant factor that mediates the loss of Lsd1 phenotype, we performed miRNA-mediated knockdown of Ovol2 in Lsd1 −/− TSCs. Remarkably, knockdown of Ovol2 completely rescues the enhanced migratory phenotype caused by the deletion of Lsd1 ( Fig. 7c ). Accordingly, knockdown of Ovol2 in wild-type cells decreases migration specifically in differentiating TSCs, while knockdown of Ovol2 in undifferentiated TSCs, which hardly express Ovol2 ( Fig. 5a,b ), does not affect migration ( Fig. 7d ). Of note, knockdown of Ovol2 does not increase Lsd1 expression ( Fig. 7c ), demonstrating that Ovol2 is a major mediator of Lsd1-controlled migration. Importantly, the ectopic expression of Ovol2 does not affect stemness and differentiation of TSCs indicated by unaltered Cdx2 , Pl1 and Gcm1 expression levels, respectively ( Supplementary Fig. 7 ). Taken together, our data demonstrate that enhanced and premature expression of Ovol2 induced by functional loss of Lsd1 accounts for the pro-migratory phenotype observed in Lsd1 −/− TSCs. 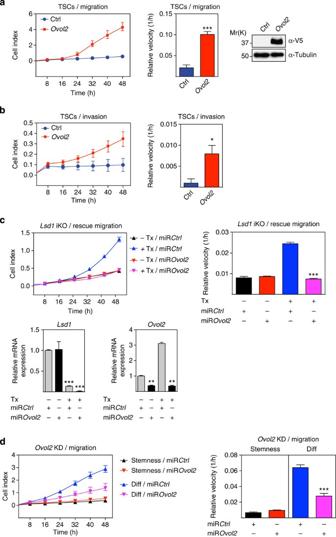Figure 7:Ovol2expression mediates increased migration and invasion ofLsd1-depleted TSCs. (a,b) Ectopically expressed Ovol2 induces increased migration (a) and invasion (b) behaviour of undifferentiated TSCs, in comparison to control-transfected (Ctrl) TSCs as monitored in real time. Ectopic expression of V5-tagged Ovol2 is controlled using western blot analysis. (c) Migration assays of undifferentiatedLsd1 iKOTSCs in the absence or presence of Tx and simultaneous miRNA-mediated knockdown demonstrate decreased migration ofLsd1-depleted TSCs uponOvol2depletion. mRNA expression levels ofOvol2andLsd1were controlled with qRT–PCR. (d) Migration assays of undifferentiated and differentiatingLsd1-proficient TSCs uponOvol2depletion in comparison to control (Ctrl) TSCs. qRT–PCR data are normalized toGapdhand represented as mean+s.e.m. Bars represent mean±s.e.m. or +s.e.m. Experiments were independently repeated at least three times in triplicate. Statistical analysis was performed using two-tailed Student’st-test. *P<0.05; **P<0.01; ***P<0.001. Figure 7: Ovol2 expression mediates increased migration and invasion of Lsd1 -depleted TSCs. ( a , b ) Ectopically expressed Ovol2 induces increased migration ( a ) and invasion ( b ) behaviour of undifferentiated TSCs, in comparison to control-transfected (Ctrl) TSCs as monitored in real time. Ectopic expression of V5-tagged Ovol2 is controlled using western blot analysis. ( c ) Migration assays of undifferentiated Lsd1 iKO TSCs in the absence or presence of Tx and simultaneous miRNA-mediated knockdown demonstrate decreased migration of Lsd1 -depleted TSCs upon Ovol2 depletion. mRNA expression levels of Ovol2 and Lsd1 were controlled with qRT–PCR. ( d ) Migration assays of undifferentiated and differentiating Lsd1 -proficient TSCs upon Ovol2 depletion in comparison to control (Ctrl) TSCs. qRT–PCR data are normalized to Gapdh and represented as mean+s.e.m. Bars represent mean±s.e.m. or +s.e.m. Experiments were independently repeated at least three times in triplicate. Statistical analysis was performed using two-tailed Student’s t -test. * P <0.05; ** P <0.01; *** P <0.001. Full size image In the present study, we analyse functions of the histone demethylase Lsd1 in the trophectoderm and identify Lsd1 as an important regulator for differentiation onset in TSCs. In the absence of Lsd1, TSCs exhibit several features of early differentiating trophoblast cells such as increased cell size, differentiation-associated changes in the gene-expression signature, and onset of cell migration and invasion. Interestingly, the premature expression of a gene signature characterizing early differentiation is not associated with the general downregulation of stemness-maintaining transcription factors such as Cdx2 and Eomes, and Lsd1 -deficient TSCs can be maintained in culture over extended periods of time. This function of Lsd1 is reminiscent to a previous report describing that Lsd1 is required for the maintenance of pluripotency in hESCs by controlling the bivalent chromatin marks at regulatory sites of early differentiation-associated genes [23] . Expression of endogenous Lsd1 decreases during hESC differentiation. Accordingly, the loss of Lsd1 in hESCs results in precocious differentiation onset. In comparison, deletion of Lsd1 in mouse ESCs does not cause premature differentiation [21] , [24] and unlike the situation in hESCs, we do not find significant changes in the expression levels of endogenous Lsd1 during the differentiation process of TSCs. One report showed that Lsd1 is required for full silencing of the stem cell programme [24] , and Foster et al. [21] proposed that Lsd1 is essential for the expression and appropriate timing of the key developmental regulators. Considering the role of Lsd1 in TSCs, it is tempting to speculate that the enzymatic activity of Lsd1 might generally act in stem cell populations to control the timely transition from stemness state to differentiation. Since the levels of Lsd1 are not altered during differentiation, Lsd1 activity might be regulated either by post-translational modifications and/or by the composition of Lsd1-interacting proteins. One prominent feature of differentiating TSCs is an increase in their migration and invasive behaviour. In our attempts to identify Lsd1-regulated genes that account for this pro-migratory behaviour, we found that premature expression of the direct target gene Ovol2 , in major parts, mediates increased migration and invasiveness of Lsd1 -deficient TSCs. During migration of Lsd1 −/− TSCs we observe reduced membrane staining for E-cadherin (Cdh1) and beta catenin (Ctnnb1), required for the formation of epithelial cell–cell adherens junctions, and increased levels of the mesenchymal marker vimentin (Vim), two hallmarks of epithelial–mesenchymal transition (EMT) ( Supplementary Fig. 3a ). In contrast to our expectation, the genome-wide expression profiling did not reveal significant changes in the majority of the typical EMT-associated regulators such as Snai1 , Twist1 or Zeb1 in Lsd1 −/− TSCs ( Supplementary Table 4 ). Thus, our data currently do not allow to unequivocally classify the aberrant migration of Lsd1 -deficient TSCs as EMT at the molecular level. Instead, we propose that Ovol2 acts as a previously unrecognized inducer of migration and cell invasion during development. Indeed, the loss-of-function phenotype of Ovol2 -deficient embryos reported by Unezaki et al. [33] already suggested that Ovol2 is required for the invasive cell behaviour of developing blood vessels and expansion of the labyrinthine layer of the placenta, leading to embryonic death around E10.5. Importantly, in our experiments Ovol2 does not seem to primarily have an impact on lineage specification of differentiating TSCs ( Supplementary Fig. 7 ) but mostly affects cellular behaviour. Interestingly, a recent study by Abbell et al. [35] reported on a similar migration phenotype of TSCs deficient for the protein kinase Map3k4 and the histone acetyltransferase CBP/p300 . These mutant TSCs concomitantly maintain properties of stemness state while showing increased migration and as such resemble features of Lsd1 -deficient TSCs [35] . Map3k4-deficient TSCs exhibit a global absence of the H2AK5ac mark, a reduction of the H2BK5ac mark and an increase in H3K9ac in comparison with wild-type cells [35] . We compared the global levels of histone acetylation in wild-type and Lsd1 −/− TSCs and found an increase in H2AK5ac and H2BK5ac marks, while the levels of H3K9ac were not altered ( Supplementary Fig. 8a ). Additionally, the data presented by Abbell et al. [35] reveal that neither Lsd1 nor Ovol2 are targets of Map3k4 and CBP/p300 , suggesting that distinct molecular pathways regulate migration during TSC differentiation. Previous reports linked Lsd1 with NuRD and CoREST complex to regulate EMT-related processes in cancer progression and in cell culture-based EMT assays [17] , [36] , [37] , [38] . More specifically, Wang et al. [17] showed that LSD1 influences the metastatic potential of breast cancer cell line MDA-MB-231. Expression profiling data from this report and our data show that OVOL2 expression is not altered after the knockdown of LSD1 in the MDA-MB-23 cell line ( Supplementary Fig. 8b ), indicating that Lsd1 controls cell migration via different, cell-context-dependent mechanisms. Interestingly, Lsd1 not only controls differentiation onset of TSCs, but also directs TSC fate. Lsd1 is required for the correct differentiation of spongiotrophoblast and trophoblast giant cells, while syncytiotrohoblast differentiation is promoted in the absence of Lsd1. This fits well to the observation of increased Ovol2 levels found in the syncytiotrophoblast of the developing placenta. It will be interesting to learn which Lsd1-regulated genes control additional aspects of early TSC differentiation, including lineage specification and proliferation control. As the most prominent feature of the Lsd1 phenotype in the early embryo, we observed a drastic reduction in the extraembryonic ectoderm and its derivatives. This reduction in placental tissues could be caused either by reduced proliferation, increased cell death or premature differentiation. Surprisingly, Lsd1 -deficient TSCs cultured in stemness-maintaining conditions do not show reduced proliferation and we could not observe increased cell death in the embryo. However, after differentiation onset, Lsd1-deficient cells show significantly reduced proliferation, possibly explaining the gross reduction in placental tissues outside of the extraembryonic ectoderm. Additionally, we cannot rule out that Lsd1 -deficient TSCs in the embryo start to prematurely differentiate, even though Lsd1 −/− TSCs can be maintained indefinitely under culture conditions. Under these culture conditions, the deletion of Lsd1 does not seem to affect responsiveness to either signals of FGF or TGFb, as demonstrated using western blot for the activated signalling mediators p-ERK and SMAD2 ( Supplementary Fig. 8c ) and maintained expression of TSC markers Cdx2 and Eomes, which depend on Fgf and TGFb signals. In summary, our functional analyses of the epigenetic regulator Lsd1 in TSCs during early stages of mouse development and in cell culture demonstrate that Lsd1 is essential for trophectoderm development by prevention of premature TSC differentiation onset including an increase in cell migration and invasion behaviour. Additionally, Lsd1 is required for directing the fate of differentiating TSCs. Thus, this study contributes to the general understanding of epigenetic modulators and their importance for the initial steps of differentiation onset and differentiation-associated cell behaviour of stem cell populations. Mice All mice were housed in the pathogen-free barrier facility of the University Medical Center Freiburg in accordance with the institutional guidelines and approved by the regional board. The targeting strategy for the conditional deletion of the first exon of Lsd1 ( Lsd1 tm1Schüle ) and the generation of Ppm1a creERT2 mice is available upon request. Tg(Sox2-cre)1Amc and Eomes tm3.1(cre)Rob mice were previously described [25] , [26] and inducible Lsd1 iKD mice were generated by introduction of the knockdown construct into the Rosa26 locus via recombinase-mediated cassette exchange [39] . The following sequences were used to knockdown Lsd1 (5′-TCCCGGATGTCACACTTCTGGAAGCTTCAAGAGAGCTTCCAGAAGTGTGACATCCTTTTTA-3′; 5′-CCTACAGTGTGAGACCTTCGAAGTTCTCTCGAAGGTCTTCACACTGTAGGAAAAATGCGC-3′). Mice were genotyped with conventional PCR using standard conditions and primers listed in Supplementary Table 5 . TSC cell culture Derivation and cultures of TSCs was performed according to published protocols [29] . In short, primary TSC lines were isolated from E3.5 blastocysts. TSCs were cultured in the absence of primary MEFs in medium supplemented with FGF4 (RD, 235-F4-025/CF, 30 ng ml −1 ) and heparin (Sigma, H3149, 1.2 μg ml −1 ). The medium contained 30 vol% TS medium (RPMI 1640, BD Biosciences, 354230), which includes 20% ES cell-qualified foetal bovine serum (Invitrogen), 1% penicillin–streptomycin (Lonza, DE17-602E), 1% glutamine (Lonza, BE17-605E), 1% sodium pyruvate (Invitrogen, 11360), 0.1 mM ß-mercaptoethanol and 70 vol% MEF-conditioned medium (collected from mitomycin C-treated (Sigma, M4287) MEFs cultured in TS medium) [40] . To induce differentiation, TSCs were cultured in TS medium in the absence of FGF4, heparin and MEF-conditioned medium. Lsd1 iKD and iKO TSCs were induced by 1 μg ml −1 doxycyclin (Ratiopharm, 576.00.01) and by 0.2 μM 4OH-tamoxifen (Sigma, H-7904), respectively. TSCs were transfected with Lipofectamine LTX according to the manufacturer’s instructions (Invitrogen). Puromycin (Sigma, P8833, 1.5 μg ml −1 ) was administrated to cells 24 h post transfection. TSCs were transfected with the following miRNA directed against mouse Ovol2 (5′-TGCTGTTTAGGTGGGACTCCAAGGAAGTTTTGGCCACTGACTGACTTCCTTGGTCCCACCTAAA-3′; 5′-CCTGTTTAGGTGGGACCAAGGAAGTCAGTCAGTGGCCAAAACTTCCTTGGAGTCCCACCTAAAC-3′) cloned into pRTS. MDA-MB-231 cells were cultured in DMEM (Lonza 12-614Q) with 10% foetal bovine serum (Invitrogen, 10270-106), 1% penicillin–streptomycin and 1% glutamine. For Lsd1 knockdown [14] cells were seeded at 3 × 10 5 cells in a 10-cm dish and transfected with 25 nM siRNA (final concentration) using Dharmafect 4 (Thermo Scientific). In situ analyses Embryos at E6.5 to E8.5 were dissected in phosphate-buffered saline (PBS) and fixed in 4% paraformaldehyde, dehydrated and embedded in paraffin. Rehydrated 5-μm sections were used for HE counterstaining, in situ hybridization [41] and immunofluorescence after antigen retrieval [42] using standard protocols. In situ hybridization analysis was carried out using a probe for Ovol2, which can be requested from the authors. For immunofluorescence, α-Cdx2 (BioGenex, MU392A-UC, 1:50), α-Eomes (Abcam, ab23345, 1:200), α-Lsd1 (no. 3544, 1:200 (ref. 14 ), α-Oct4 (Santa Cruz, C-10, 1:50), α-Vimentin (Sigma, V-2258, 1:100), α-Cdh1 (BD transduction lab, 610182, 1:100) and α-Ctnnb1 (BD transduction lab 610154, 1:100) antibodies were used. Specific staining was monitored by hybridization to unrelated mouse (sc-2025), rabbit (sc-2027) and rat (sc-2026) IgG (Santa Cruz) diluted to the same concentration as corresponding primary antibodies. Alexa Fluor-488 goat α-rabbit IgG and Alexa Fluor 546 goat α-mouse IgG (Molecular Probes, 1:1,000) were used as secondary antibodies and DAPI (2 μg ml −1 ) for counterstaining of nuclei. F-actin was stained with Alexa Fluor-488 Phalloidin (Invitrogen, A12379). Staining was documented with a confocal microscope (Leica SP2AOBS). Western blot analysis Experiments were performed as described [14] . Briefly, cells were lysed in SC buffer and 30 μg of protein extract supernatant was used for western blots. The following antibodies were used: α-beta Actin (Sigma, A1978, 1:15,000), α-Cdx2-88 (BioGenex, MU392A-UC, 1:200), α-Eomes (Abcam, ab23345, 1:1,000), α-p-ERK1/2 (Cell Signaling, 9101, 1:1,000), α-ERK1/2 (Cell Signaling, 46951, 1:1,000), α-H2A (Abcam ab13923, 1:1,000), H2AK5ac (Millipore, 1:1,000), α-H2B (Santa Cruz, sc-10808, 1:200), α-H2BK5ac (Robert Schneider, 1:1,000), α-H3 (Abcam, ab1791, 1:5,000), α-H3K9ac (Diagenode, pAb-ACHAHS-044, 1:500), α-Lsd1 (Schüle laboratory 3583, 1:2,000 (ref. 14 )), α-Pl1 (Santa Cruz, P-17, 1:1,000), α-p-Smad2 (Cell Signaling, 3101, 1:1,000), α-Smad2/3 (BD Transduction Lab, 610843, 1:1,000), α-alpha-tubulin (Sigma, T6074, 1:10,000) and α-V5 (Invitrogen, R960-25, 1:1,000), α-Flag M2 (Sigma, F3165, 1:2,500), α-Ovol2 (Schüle laboratory 8053, 1:1,000). Histones were purified according to the manufacturer’s instruction (Active Motif; Histone Purification Kit, 40025). All full-scan western blots are provided in Supplementary Fig. 9 . Plasmids Expression plasmids for Ovol2 , Lsd1 and Lsd1 Mut were generated by LRII recombination according to the supplier (Gateway, Invitrogen) using entry clones (GeneCopoeia; GC-Mm13121-CF; accession number NM_026924.3; pENTR-Flag-Lsd1, pENTR-Flag-Lsd1 Mut [30] , Schüle laboratory) and a puromycin-selectable and doxycyclin-inducible pRTS plasmid [43] , modified to contain a Gateway cassette, V5 and His tags. RNA extraction and quantitative RT–PCR RNA isolation and quantitative PCR with reverse transcription were performed as described [14] . Gapdh was used for normalization and data were related to undifferentiated wild-type TSCs. For normalization of expression in MDA-MB-231 cells, GAPDH , HPRT1 and POLR2A were used and data were related to cells treated with control siRNA. Experiments were repeated in triplicate three times. Primers are shown in Supplementary Table 5 . TaqMan gene expression assay (Life Technologies; no. 4331182) was used to determine Gcm1 expression. Cell culture assays Prior to the experiment, Lsd1 iKO and iKD TSCs were treated for 8 days with Dox or Tx, respectively. Proliferation assays were performed essentially as described [14] by seeding 3 × 10 3 and 6 × 10 3 cells in 96-well plates in TSC stemness or differentiation culture medium, respectively. The cell proliferation enzyme-linked immunosorbent assay (ELISA) BrdU Colorimetric Assay (Roche) was performed according to the manufacturer’s instructions after 24, 48 and 72 h. The experiments were repeated in quadruplicate three times. Cell migration and invasion were monitored using the xCelligence system (Roche). For invasion, transwell chamber filters (Roche) were coated with matrigel (BD Biosciences, 354230) diluted 1:20 in RPMI-1640 medium. Lsd1 iKD or iKO TSCs were seeded at 1 × 10 5 cells into transwell in TSC culture medium in the presence or absence of FGF4 and heparin. TSCs were cultured 24 h before and during the experiment in the presence of 10 μM Lsd1 inhibitors substance 1 (2-[(2-{4-[4-fluoro-2-(trifluoromethyl)phenyl]phenyl}cyclopropyl)amino]-1-(4-methylpiperazin-1-yl)ethan-1-one) [32] , substance 2 (trans-N-[1-(2,3-dihydro-1,4-benzodioxin-6-yl)ethyl]-2-phenylcyclopropan-1-amine) [31] , substance 3 (trans-N-[(2-methoxypyridin-3-yl)methyl]-2-phenylcyclopropan-1-amine) [31] or DMSO. Cell indices were automatically recorded every 15 min. For visualization, invaded cells were fixed with 4% paraformaldehyde for 5 min on transwell membrane and stained with 0.4% crystal violet for 20 min. FACS Cell size of TSCs was analysed using the Forward Scatter of the FACScalibur (Becton Dickinson). Data were plotted in a single dimension using the CellQuestPro software. For proliferation assays, 2 × 10 5 TSCs were seeded and cultured for 48 h under stemness-maintaining or differentiation conditions. Cell number was determined by addition of AccuCheck counting beads (Invitrogen) to each sample using the FACScalibur for detection. cDNA microarray and bioinformatics Before the start of the experiment, Lsd1 iKO TSCs were treated with Tx for 8 days. Cells were harvested before 2 and 4 days after induction of differentiation. RNA was isolated using Trizol (Invitrogen) according to the supplier’s protocol, DNaseI-treated (Promega) and quality controlled with 2100 Bioanalyzer (Agilent) analysis. A total of 10 μg RNA for each sample was used for reversed transcription. The cDNA was hybridized to GeneChip MG-430_2.0 arrays (Affymetrix). Expression values were normalized using the RMA algorithm performed with R and Bioconductor software. Further analysis was performed using the Analyst 2.2 software (Genedata, Basel; Switzerland) and DAVID [44] , [45] . A principal component analysis and hierarchical clustering were used to exclude outliers from further analysis. ChIP ChIP experiments and quantitative PCR were performed essentially as described [14] . For performing ChIPs, Lsd1 iKO TSCs were cultured in the presence or absence of Tx and were harvested before and 4 days after induction of differentiation. Cells were washed with PBS and crosslinked with 1% formaldehyde in PBS for 20 min at 4 °C. Cells were then rinsed twice with ice-cold PBS, collected into PBS and centrifuged for 5 min at 2,500 r.p.m. at 4 °C. The pellets were then resuspended in 0.3 ml of lysis buffer (0.1% SDS, 10 mM EDTA, 50 mM Tris-HCl, pH 8.0 and 1% protease inhibitor cocktail ( Roth )) and sonicated for 20 min using a Bioruptor (Diagenode; level H, interval on/off: 0.5), followed by centrifugation for 10 min at maximal speed at 4 °C. Supernatants were collected and diluted in dilution buffer (1% Triton X-100, 2 mM EDTA, 150 mM NaCl and 20 mM Tris-HCl, pH 8.0) followed by immunoclearing with 2 μg sheared fish sperm DNA and protein A-Sepharose CL-4B ( Amersham Biosciences ) (50 μl of 50% slurry in 10 mM Tris-HCl, pH 8.0 and 1 mM EDTA) for 2 h at 4 °C. Immunoprecipitation was performed overnight at 4 °C with specific antibodies (250 μg DNA using 5 μg antibody). After immunoprecipitation, 50 μl protein A-Sepharose and 2 μg fish sperm DNA were added, and incubation was continued for another 1 h. Sepharose beads were washed sequentially for 10 min each in TSE I (0.1% SDS, 1% Triton X-100, 2 mM EDTA, 150 mM NaCl, 20 mM Tris-HCl, pH 8.0), TSE II (0.1% SDS, 1% Triton X-100, 2 mM EDTA, 20 mM Tris-HCl, pH 8.0, 500 mM NaCl) and Buffer III (0.25 M LiCl, 1% NP-40, 1% deoxycholate, 1 mM EDTA, 10 mM Tris-HCl pH 8.0). Beads were then washed three times with TE buffer (10 mM Tris-HCl, pH 8.0 and 1 mM EDTA) and extracted with 100 μl of 1% SDS, 0.1 M NaHCO3. Eluates were pooled and heated at 65 °C overnight to reverse the crosslinking. DNA fragments were purified with a DNA purification kit (QIAquick PCR purification Kit, Qiagen GmbH). For qPCR, 2 μl out of 50 μl DNA extract were used. qPCR analyses were performed using the LightCycler system (Roche) and ABsolute SYBR green ROX Mix (Thermo Scientific). Immunoprecipitations were performed with rbIgG (Diagenode, kch-504-250, lot DW0502), α-Lsd1 (no. 3544 (ref. 14 )), α-H3K4me1 (Active Motif, 39297, lot21008001), α-H3K4me2 (Diagenode, CS-035-100, lot A391-001), α-H3K4me3 (Abcam, ab8580, lot GR33087-1), α-H3K9me1 (Millipore, 07-450, lot DAM1680820), α-H3K9me2 (Active Motif, 39753, lot 06710001), α-H3K9me3 (Millipore, 07-442, DAM1687549), α-H3K27me3 (Millipore, 07449, lot DAM1514011), α-PolII (Santa Cruz, N-20, sc-899, lot no. C1413) and α-H3 (Abcam, ab1791, lot GR15960-2) antibodies on protein A-Sepharose 4B (GE-Healthcare). The primers for quantitative PCR are shown in Supplementary Table 6 . Statistical analysis If not otherwise stated, significance was calculated using an unpaired t -test. Data are calculated as mean±s.e.m. or +s.e.m. Experiments were repeated at least three times in triplicate. Accession codes: All microarray data are deposited at the GEO database repository under accession number GSE38277 . How to cite this article: Zhu, D. et al. Lysine-specific demethylase 1 regulates differentiation onset and migration of trophoblast stem cells. Nat. Commun. 5:3174 doi: 10.1038/ncomms4174 (2014).